Atomic-scale dynamic process of deformation-induced stacking fault tetrahedra in gold nanocrystals Stacking fault tetrahedra, the three-dimensional crystalline defects bounded by stacking faults and stair-rod dislocations, are often observed in quenched or irradiated face-centred cubic metals and alloys. All of the stacking fault tetrahedra experimentally observed to date are believed to originate from vacancies. Here we report, in contrast to the classical vacancy-originated ones, a new kind of stacking fault tetrahedra formed via the interaction and cross-slip of partial dislocations in gold nanocrystals. The complete atomic-scale processes of nucleation, migration and annihilation of the dislocation-originated stacking fault tetrahedra are revealed by in situ high-resolution observations and molecular dynamics simulations. The dislocation-originated stacking fault tetrahedra can undergo migration and annihilation due to mechanical loading in a manner that is not expected in bulk samples. These results uncover a unique deformation mechanism via dislocation interaction inside the confined volume of nanocrystals and have important implications regarding the size effect on the mechanical behaviour of small-volume materials. Plastic deformation in metals and alloys is governed by the generation and evolution of defects of point, line, plane and volume types [1] , [2] . Among these defects, stacking fault tetrahedra (SFT), bounded by stacking faults (SFs) and stair-rod dislocations, are peculiar types of volume defect typically found in face-centred cubic (FCC) crystals with low stacking fault energy [1] , [3] . Generally, SFT can be introduced by three methods, that is, quenching, high-energy particle irradiation and plastic deformation [3] , [4] , [5] , [6] , [7] , [8] . In 1959, Silcox and Hirsch [4] first observed SFT in quenched gold (Au). They proposed that SFT were formed from the Frank dislocation loops generated by collapsed vacancy clusters, which further dissociated through the Silcox–Hirsch mechanism [1] , [4] to produce the three-dimensional (3D) SFT. Since then, extensive studies have been conducted on the vacancy-originated SFT in quenched, irradiated or plastically deformed bulk FCC crystals [3] , [4] , [5] , [6] , [7] , [8] , [9] , [10] , [11] , [12] , [13] , [14] , [15] , [16] , [17] , [18] , [19] , [20] , [21] , [22] , [23] , [24] . However, whether the SFT can be possibly initiated by dislocations without the aid of vacancies remain largely unexplored. If possible, how do SFT form, migrate and annihilate, particularly at the nanoscale level? It is well known that the smaller tends to be stronger [25] , [26] and the free surface in nano-sized crystals acts as an effective source of dislocations [27] , [28] , [29] . However, surface nucleation only leads to a weak size effect on the strength of nanocrystals [27] , [30] , for example, the predicted logarithmic scaling of strength versus nanopillar/nanowire diameter as opposed to the measured power law scaling. Hence, the widely observed size effect is generally believed to arise from dislocation interactions inside nanocrystals. Moreover, the study of plasticity in nanocrystals has until now been focused on one-dimensional (1D) (dislocation) and two-dimensional (2D) (grain boundary) defects [27] , [28] , [29] , [31] , [32] , [33] . It remains unclear whether higher-order defects, such as the 3D volume defect of SFT, can be generated inside the confined volume of nanocrystals by pure mechanical deformation. Furthermore, as the sources of partial dislocation are abundant at the surface [27] , [28] , [29] , they might facilitate the interactions between partials and SFT in the small volume of nanocrystals. It is thus expected that the dynamic evolution of the SFT might be uniquely mediated by SFs in the nanoscale regime. However, because of technical difficulties in controlling the samples at the nanoscale level, it has been a challenge to directly explore the dislocation interaction, as well as the formation and evolution of higher order defects, in small-volume nanocrystals. Here we report the first direct visualization of the formation and evolution of the deformation-induced SFT via dislocation interactions during in situ tensile testing of Au nanocrystals with high-resolution transmission electron microscopy (HRTEM). Aided by large-scale molecular dynamics (MD) simulations, we show that the SFT can be produced in nanocrystals directly through dislocation interactions. The presence of vacancies that is critical for the initiation of SFT in the bulk is no longer a pre-requisite for the SFT formation in the nanoscale. We hence term the SFT formed in the nanocrystals as ‘dislocation-originated’ SFT, specifically because of its origin being solely controlled by dislocation interaction events. Our finding, to our knowledge, is the first ever instance of SFT formation reported in the nanoscale regime. Moreover, we observe the migration and annihilation of the dislocation-originated SFT, which are proved to be a direct outcome of dislocation–SFT interactions. 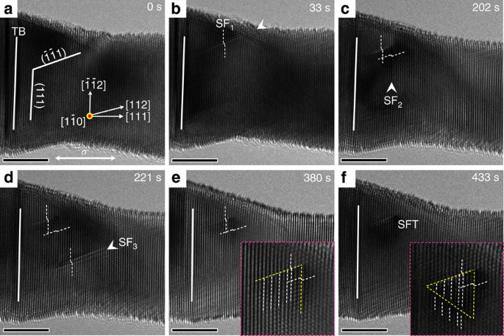Figure 1: Formation of dislocation-originated SFT. (a) Crystallographic orientation of the Au nanowire embedded with a TB. The nanowire diameter is about 16 nm. (b–f) Sequential HRTEM images showing the evolution of dislocation structure and the formation of a dislocation-originated SFT via the interactions of partial dislocations under [111] tensile loading. Upon tensile loading, the partial dislocations with SFs nucleate sequentially from the free surface on the equivalent inclined {111} planes and interact with each other, forming a wedge (c) and then a zigzag (d) dislocation structure. (e) At 380 s, SF3propagates and annihilates at the free surface, leaving behind the wedge structure. The inset shows the enlarged HRTEM image of the wedge structure (yellow dashed line). (f) The wedge dislocation structure further evolves into a triangular defect, which is identified to be an SFT. The inset marks out the SFT by a yellow triangle. Scale bar, 5 nm. Formation of Dislocation-originated SFT by Dislocation Interactions Figure 1 and Supplementary Movie 1 show the formation of a dislocation-originated SFT through the interactions of partial dislocations in an Au nanowire. The Au nanowire is 16 nm in diameter and contains a growth twin boundary (TB). It is loaded along the [111] direction and viewed along the direction ( Fig. 1a ). During tensile deformation, the partial dislocation typically nucleates from the free surface and moves into the Au nanowire ( Fig. 1b ), which is consistent with our previous experimental observations [28] , [29] . It is observed that several SFs nucleate sequentially at different sites of the free surface. They glide on the equivalent, inclined {111} planes (denoted as SF 1 , SF 2 and SF 3 , respectively) and interact with each other inside the Au nanowire, forming a wedge and then a zigzag dislocation structure ( Fig. 1c,d ). Such interactions between the SFs are the first step of the formation of dislocation-originated SFT. As the tensile load increases, SF 3 starts to move and eventually annihilates at the free surface, leaving behind a wedge structure between SF 1 and SF 2 ( Fig. 1e ). This wedge structure involves both SF 1 and SF 2 with a 1/6<110>-type stair-rod dislocation at the intersection between the two SFs (inset in Fig. 1e ). It further evolves under the applied load, resulting in a 2–3-nm-sized triangular defect (as indicated by the yellow triangle in the inset of Fig. 1f ). Such a triangular defect is identical to the projected view of SFT along the direction in both its shape and geometric angles ( Supplementary Fig. S1a,b ). Moreover, the morphology of this triangular defect appears to be the same as that of the vacancy-originated SFT reported in the literature [6] , [12] , [34] . Figure 1: Formation of dislocation-originated SFT. ( a ) Crystallographic orientation of the Au nanowire embedded with a TB. The nanowire diameter is about 16 nm. ( b – f ) Sequential HRTEM images showing the evolution of dislocation structure and the formation of a dislocation-originated SFT via the interactions of partial dislocations under [111] tensile loading. Upon tensile loading, the partial dislocations with SFs nucleate sequentially from the free surface on the equivalent inclined {111} planes and interact with each other, forming a wedge ( c ) and then a zigzag ( d ) dislocation structure. ( e ) At 380 s, SF 3 propagates and annihilates at the free surface, leaving behind the wedge structure. The inset shows the enlarged HRTEM image of the wedge structure (yellow dashed line). ( f ) The wedge dislocation structure further evolves into a triangular defect, which is identified to be an SFT. The inset marks out the SFT by a yellow triangle. Scale bar, 5 nm. 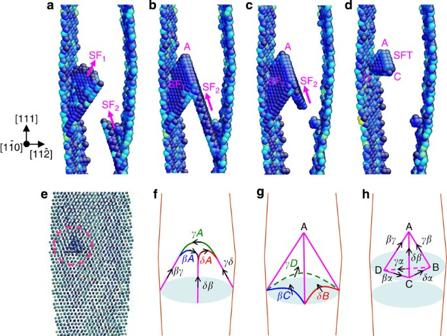Figure 2: Formation of dislocation-originated SFT in MD simulations. The Au nanowire is loaded in the [111] direction. (a) A leading partial with trailing SF1nucleates from the free surface on the (1) plane under tensile loading. (b) Two new SFs, SF2and SF3, nucleate on the (1) and (1) plane, respectively, and intersect with SF1, forming the initial open-SFT. Note that SF3is covered visually by SF1and SF2and thus cannot be seen directly. (c) The nucleation of trailing partials sweeps out part of the SFs, thus removing the trails of the initial open-SFT. (d) The closed SFT finally forms by dislocation cross-slip. (e) Projection view of the closed SFT along the <110> direction. (f–h) Schematic illustration of the detailed dislocation processes during the SFT formation. Full size image Figure 2 shows the formation of dislocation-originated SFT via dislocation interactions in an Au nanowire, as realized in our MD simulations. The Au nanowire is subjected to tensile loading along the [111] axial direction. Similar to our experimental observation, a leading partial dislocation of 1/6<112>-type and of a Schmid factor of 0.31 (denoted as βA in Fig. 2f ) is seen to nucleate from the nanowire surface; it propagates on the plane, leaving SF 1 behind ( Fig. 2a ). Subsequently, two new partial dislocations, denoted as δA and γA (and with the same Schmid factor of 0.31) are triggered on the and planes, respectively, enclosing SF 2 and SF 3 ( Fig. 2b,f ). Note that SF 3 is covered visually by SF 1 and SF 2, and thus cannot be seen in Fig. 2b,c . Partials of δA and γA propagate into the nanowire and lock with βA , forming three 1/6<110>-type sessile stair-rod dislocations, denoted as βγ , δβ and γδ in Fig. 2f (and Supplementary Note 1 ). These sequential dislocation nucleation and interaction events create an initial ‘open-SFT’ with only three completed faces ( Fig. 2b ). Under further tensile loading, trailing partial dislocations βC , δB and γD , which have a Schmid factor of 0.16, nucleate as in Fig. 2g , the propagation of which eliminates a part of the SFs on each of the three faces of the open-SFT ( Fig. 2c,g ), thus removing the trails of the initial open-SFT. A closed SFT finally forms via the cross-slip of one of the trailing partials into the open (111) plane, producing SF 4 that constitutes the base of the closed SFT; the three 1/6<110>-type sessile dislocations βα , δα and γα enclose the base of the closed SFT ( Fig. 2d,h and Supplementary Fig. S2 ). Figure 2e shows the projected image of the SFT in Fig. 2d as viewed along the <110> direction, which is same as the experimental observation under HRTEM in Fig. 1f (as compared in Supplementary Fig. S1c–e ). The simulation result is consistent with our experimental observation in that the SFT are produced directly by a sequence of partial dislocation nucleation and interaction events in nanocrystals, which is hence different from the vacancy-originated mechanism of SFT formation in bulk materials. Figure 2: Formation of dislocation-originated SFT in MD simulations. The Au nanowire is loaded in the [111] direction. ( a ) A leading partial with trailing SF 1 nucleates from the free surface on the ( 1) plane under tensile loading. ( b ) Two new SFs, SF 2 and SF 3 , nucleate on the ( 1 ) and (1 ) plane, respectively, and intersect with SF 1 , forming the initial open-SFT. Note that SF 3 is covered visually by SF 1 and SF 2 and thus cannot be seen directly. ( c ) The nucleation of trailing partials sweeps out part of the SFs, thus removing the trails of the initial open-SFT. ( d ) The closed SFT finally forms by dislocation cross-slip. ( e ) Projection view of the closed SFT along the <110> direction. ( f – h ) Schematic illustration of the detailed dislocation processes during the SFT formation. Full size image The structure of the dislocation-originated SFT is compared with the vacancy-originated SFT. 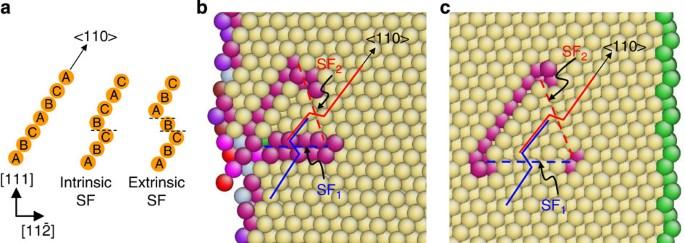Figure 3: Crystallographic structure of the SFT. (a) Schematic representation of the intrinsic and extrinsic stacking faults in terms of the A/B/C atomic layer stacking, as well as the single and double kinking (faults) along the close-packed direction of <110>. (b) {110} cross-section of a dislocation-originated SFT, with atoms coloured by their coordination numbers. (c) Same as (b) except for a vacancy-originated SFT formed via the Silcox–Hirsch mechanism. Figure 3a presents the schematics of intrinsic and extrinsic SFs by using a line of atoms with the single and double faults of stacking along the close-packed direction of <110>. With such schematics as reference, it is evident that the SFs (for example, SF 1 and SF 2 ) in a dislocation-originated SFT are of the intrinsic type ( Fig. 3b ), each of which involves only one faulted plane of stacking. In Fig. 3c , a vacancy-originated SFT is ‘artificially’ created in a nanowire by relaxing a triangular vacancy loop (that is, a Frank loop) [12] , [17] . Each of the SFs also involves only one faulted plane of stacking, and thus is of the intrinsic type. The minor differences in colour between the two types of SFT arise owing to the fact that the former is subjected to a large tensile stress, whereas the latter is stress-free. Comparison between the two types of SFT proves that the dislocation-originated SFT is structurally equivalent to the vacancy-originated SFT. However, the dislocation-originated SFT can have an important role in controlling the plasticity of FCC metallic nanostructures (see the Discussion section). Figure 3: Crystallographic structure of the SFT. ( a ) Schematic representation of the intrinsic and extrinsic stacking faults in terms of the A/B/C atomic layer stacking, as well as the single and double kinking (faults) along the close-packed direction of <110>. ( b ) {110} cross-section of a dislocation-originated SFT, with atoms coloured by their coordination numbers. ( c ) Same as ( b ) except for a vacancy-originated SFT formed via the Silcox–Hirsch mechanism. Full size image Migration of Dislocation-originated SFT Similar to the Lomer–Cottrell lock, the SFT is bounded by SFs and stair-rod dislocations [1] and is usually sessile. In nanocrystals, however, the SFs are frequently nucleated from the surface and could induce migration and annihilation of the dislocation-originated SFT by dislocation–SFT interactions. 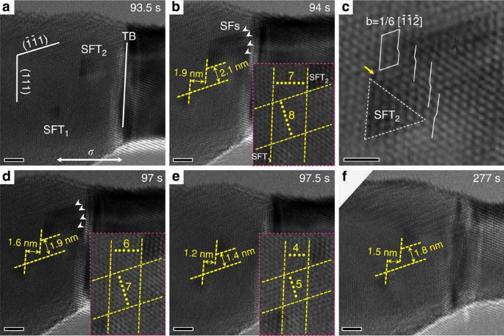Figure 4: Migration of dislocation-originated SFT during deformation. (a) Under tensile loading, two dislocation-originated SFT (SFT1and SFT2) are produced sequentially. (b) Upon further deformation, a group of partial dislocations (indicated by the white arrows) nucleate from the TB and interact with SFT2. (c) Structure of the partial dislocation group, which consists of four parallel leading partials with SFs. The yellow arrow indicates the strain contrast induced by dislocation–SFT2interaction. (d–f) The dislocation group drives SFT2to migrate, as indicated by the changes of distance and atomic layers between SFT1and SFT2on the (111) and (1) plane, respectively. Insets in (b) and (d,e) are the changes of atomic layers between SFT1and SFT2on the (111) and (1) plane, respectively. Scale bar in (a,b,d–f), 2 nm; Scale bar in (c), 1 nm. Figure 4 and Supplementary Movie 2 show the migration of a dislocation-originated SFT during the tensile deformation of an Au nanowire. In this case, two dislocation-originated SFT (SFT 1 and SFT 2 ) are produced sequentially via partial dislocation interactions ( Fig. 4a ). Upon further loading, a group of partial dislocations, which consists of four leading partials on adjacent planes ( Fig. 4c ), nucleates from the TB at a nucleation stress of about 2.3 GPa ( Supplementary Fig. S3 ) and interacts with SFT 2 ( Fig. 4b ). The dislocation group drives the migration of SFT 2 along the [00 ] direction, which can be seen from the changes in the distance (or the number of atomic layers) between SFT 1 and SFT 2 ( Fig. 4b–f and Supplementary Fig. S4 ). In the beginning, the measured distance between the two SFT on the (111) and ( 1) planes is, respectively, 1.9 and 2.1 nm ( Fig. 4b ), corresponding to seven and eight atomic layers (inset in Fig. 4b ). Subsequently, the interaction between the dislocation group and SFT 2 reduces the distance between the two SFTs ( Fig. 4d ). Finally, after the dislocation group is annihilated at the free surface, the distance between the two SFT decreases, respectively, to 1.2 and 1.4 nm on the (111) and ( 1) planes ( Fig. 4e ), corresponding to four and five atomic layers (inset in Fig. 4e ). The measured changes in the distance between the two SFT match well with the distance between the corresponding atomic layers. Interestingly, the distance between the two SFT increases after a further increase in tensile loading ( Fig. 4f ). It is worth pointing out that the size and shape of SFT 2 remain unchanged before and after its migration ( Supplementary Fig. S5 ). Figure 4: Migration of dislocation-originated SFT during deformation. ( a ) Under tensile loading, two dislocation-originated SFT (SFT 1 and SFT 2 ) are produced sequentially. ( b ) Upon further deformation, a group of partial dislocations (indicated by the white arrows) nucleate from the TB and interact with SFT 2 . ( c ) Structure of the partial dislocation group, which consists of four parallel leading partials with SFs. The yellow arrow indicates the strain contrast induced by dislocation–SFT 2 interaction. ( d – f ) The dislocation group drives SFT 2 to migrate, as indicated by the changes of distance and atomic layers between SFT 1 and SFT 2 on the (111) and ( 1) plane, respectively. Insets in ( b ) and ( d , e ) are the changes of atomic layers between SFT 1 and SFT 2 on the (111) and ( 1) plane, respectively. Scale bar in ( a , b , d – f ), 2 nm; Scale bar in ( c ), 1 nm. Full size image The migration of dislocation-originated SFT can, in principle, result from thermal or mechanical activation. Migration of dislocation loop and vacancy cluster has been observed in irradiated or quenched metals [34] , [35] , [36] , the reason for which is attributed to thermal activation [36] . In the present experiment, thermal activation is unlikely, as the migration is only observed when a group of dislocations interact with the SFT. Therefore, we attribute the migration of SFT to the activation by mechanical stress that leads to the dislocation–SFT interactions. It is known that due to applied loads, the vacancy-originated SFT can be sheared or distorted by interactions with dislocations [17] , [18] , [19] , [20] , which could result in the movement of the apex atoms of SFT to new positions [17] and thus produce ledges on SFT [20] . The migration of these ledges by the absorption of vacancies or atoms can cause the growth or shrinkage of the vacancy-originated SFT [24] , [37] . Similarly, the gliding dislocation upon interaction with the dislocation-originated SFT can produce ledges on the side of SFT for a single dislocation–SFT interaction event ( Supplementary Fig. S6 ). As a result, the SFT can effectively migrate via simultaneous interaction events with multiple dislocations. Moreover, the relatively large surface-to-volume ratio in nanocrystals, as opposed to their bulk counterparts, could promote the SFT migration by feeding more SFs from the fertile surface nucleation sites. Additionally, it should be noted that the movement of SFT is distinct from the climb or glide process of dislocation under mechanical loading. The dislocations can climb or glide by themselves under external loading, whereas the SFT cannot move by itself and its migration must be driven by the dislocations through dislocation–SFT interactions. Annihilation of Dislocation-originated SFT The annihilation of dislocation-originated SFT is also observed by our in situ experiment ( Fig. 5 and Supplementary Fig. S7a,c ). The pristine Au nanocrystal in Fig. 5 is created by cold welding between two Au nanostructures [38] . Interestingly, SFT 1 is observed in the pristine Au nanocrystal right after cold welding ( Fig. 5a ), which indicates the occurrence of plastic deformation during the cold welding process. Generally, when two nanostructures come into contact, a large mechanical stress could be induced at the contact zone owing to the mismatch of geometry and orientation, which can result in the so-called dislocation-mediated pseudoelastic deformation if the contact surface is atomically flat [39] . In our experiment, however, the surfaces of the two nanostructures are not atomically flat ( Fig. 5a ), resulting in residual dislocations or SFT upon contact. Moreover, because of the relatively low strain rate of cold welding and the large image stress associated with a small sample size, supersaturation of vacancies is unlikely in the cold-welding process and hence SFT 1 should be of the dislocation-originated type. 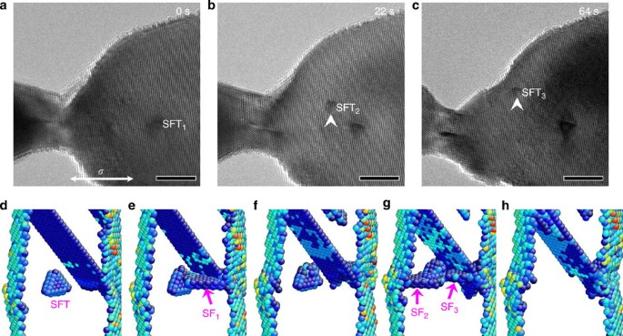Figure 5: Annihilation of dislocation-originated SFT under tensile deformation. (a–c) Sequential HRTEM images showing the annihilation of a dislocation-originated SFT induced by deformation. (a) SFT1is observed in the pristine nanocrystal after cold welding. (b) Upon tensile loading, SFT2is produced near SFT1. (c) Further deformation leads to the annihilation of SFT2and nucleation of SFT3. Scale bar in (a–c), 5 nm. (d–h) MD snapshots showing the annihilation of a dislocation-originated SFT by dislocation–SFT interactions. (d) A closed SFT formed near a TB in the Au nanowire. (e,f) A partial dislocation with SF1makes an edge-on interaction with the SFT, and shears and distorts the closed SFT. (g–h) Partial dislocations with SF2and SF3nucleate subsequently, lead to the complete annihilation of the SFT. Figure 5: Annihilation of dislocation-originated SFT under tensile deformation. ( a – c ) Sequential HRTEM images showing the annihilation of a dislocation-originated SFT induced by deformation. ( a ) SFT 1 is observed in the pristine nanocrystal after cold welding. ( b ) Upon tensile loading, SFT 2 is produced near SFT 1 . ( c ) Further deformation leads to the annihilation of SFT 2 and nucleation of SFT 3 . Scale bar in ( a – c ), 5 nm. ( d – h ) MD snapshots showing the annihilation of a dislocation-originated SFT by dislocation–SFT interactions. ( d ) A closed SFT formed near a TB in the Au nanowire. ( e , f ) A partial dislocation with SF 1 makes an edge-on interaction with the SFT, and shears and distorts the closed SFT. ( g – h ) Partial dislocations with SF 2 and SF 3 nucleate subsequently, lead to the complete annihilation of the SFT. Full size image Upon mechanical loading, a new SFT (SFT 2 ) is produced near SFT 1 ( Fig. 5b ). However, further deformation leads to the annihilation of SFT 2 and nucleation of SFT 3 ( Fig. 5c ). As the SFT 2 disappears fast (in <0.5 s), the details of annihilation are not captured during in situ experiment. However, the SF trace left indicates that the annihilation of SFT is mediated by dislocation–SFT interactions ( Supplementary Fig. S7a,c ). MD simulations ( Fig. 5d–h ) further prove that the annihilation of dislocation-originated SFT is indeed a dislocation-mediated process, which is similar to that found for the vacancy-originated SFT in the bulk [13] , [14] , [15] , [16] , [17] , [18] , [19] . Figure 4d shows a closed dislocation-originated SFT near a TB inside the nanowire. Under tensile loading, a partial dislocation loop enclosing SF 1 nucleates on (111) plane and makes an edge-on interaction with the SFT at the third atomic layer of the SFT from its apex. The closed SFT is sheared and distorted ( Fig. 5e,f ). This event is followed by similar events of newly nucleated partial dislocations shearing the closed-SFT ( Fig. 5g,h ). The Shockley partial dislocation with the trailing SF 2 nucleates and interacts with the 1/6<110>-type sessile stair-rod dislocations constituting the basal plane of the SFT. These processes lead to the formation of new 1/6<112>-type Shockley partials that would be expected to glide on the tetrahedral planes of the SFT and partially remove the SFs, as has been reported for the SFT using MD simulations [17] . However, what we observe for the SFT in the nano-sized sample is its complete destruction ( Fig. 5h ) due to the SFs intersecting at its base and/or above (SF 2 and SF 3 in Fig. 5g ), instead of only a partial destruction as in the bulk samples [15] , [19] . Moreover, as the free surface in the sub-20-nm nanocrystal serves as an efficient nucleation source of dislocations, it could thus have an important role in the annihilation of SFT by providing nucleated dislocations. SFT have usually been classified as a vacancy-originated volume defect in quenched or irradiated metals and alloys [1] , [3] , [4] , [5] , [6] . However, it is unlikely that the SFT observed in the Au nanocrystals of this work are vacancy-originated. First, a high density of vacancies is required to nucleate the vacancy-originated SFT, which is often present in quenched or irradiated metals [1] , [3] , [4] , [5] but is hardly achievable in our nano-sized metallic samples. Second, there are two possible factors regarding the electron beam effect, that is, knock-on displacement and beam heating. For the knock-on displacement to occur, the threshold electron energy for Au is 1,320 KeV [40] . The 300-KV acceleration voltage used in our experiments is therefore insufficient to produce such kind of beam damage [28] . For the beam-heating issue, the thermal conductivity of Au is high (300 W mK −1 ) and the two ends of Au nanowires are, respectively, connected to an Au substrate and an Au probe with sizes much larger than the samples. Considering the low beam current applied in our experiments (80~100 A cm −2 ) and the fact that both the Au substrate and the probe act as the effective heat sinks, the temperature rise induced by beam heating should be negligible in the sample [28] , [41] . More importantly, SFT are also observed to form during deformation without any beam irradiation and beam-induced temperature rise ( Supplementary Fig. S8 ), which further supports the conclusion that the SFT observed during plastic deformation is dislocation-originated and not vacancy-originated. Therefore, the beam irradiation and heating would have little influence on the SFT formation and the dislocation–SFT interactions. Additionally, although vacancy clusters and vacancy-originated SFT can be generated by plastic deformation, high strain rates are required [10] , [11] . In our experiments, the strain rate employed is relatively low and sufficient vacancies cannot be produced by plastic deformation alone. Even if a smaller number of deformation-induced vacancies may exist, they could easily escape the nanocrystal from its free surface owing to the large image stress associated with the small crystal size and the low strain rate employed, rather than condense into vacancy clusters inside the Au nanocrystal. Therefore, the observed SFT likely result from the interactions of partial dislocations, and our large-scale MD simulations lend a direct support to this mechanism. On the basis of these considerations, we believe that the formation, migration and annihilation of the dislocation-originated SFT are revealed for the first time in sub-20-nm nanocrystals. It is generally recognized that the surface-nucleated dislocations initiate the plastic deformation in nano-sized crystals [27] , [28] , [29] . The partial dislocations nucleated on the equivalent, inclined {111} planes can strongly interact with each other inside the small volume of Au nanocrystals, resulting in the stair-rod dislocations and nano-sized dislocation-originated SFT. We have frequently observed the dislocation-originated SFT during the deformation of Au nanocrystals with different sample sizes and loading conditions in both experiments and MD simulations ( Supplementary Figs S7–S9 and Supplementary Table S1 ). Hence, the formation and evolution of SFT should be considered as an important deformation mechanism at this length scale. Moreover, both SFT formation and dislocation–SFT interaction can contribute to the strain hardening of small-volume samples ( Supplementary Fig. S10 ). Nanocrystals are known to have limited strain hardening because of the lack of sufficient hardening obstacles (dislocations or other defects) and the easy annihilation of dislocations at the surface owing to the large image stress [28] , [29] , [42] . In contrast, the formation of dislocation-originated SFT is a novel mechanism by which the nanocrystal could achieve finite amounts of inherent hardening. In addition, SFT act as strong obstacles to the motion of other dislocations (as shown in Fig. 3 ) and contribute to further hardening. Furthermore, our results indicate that the SFT formation is not limited to the specific set of dimensions of the simulated nanowire, and the size of SFT formed depends on the sample size ( Supplementary Note 2 ). Dislocation-originated SFT are also formed in a deformed Cu nanowire following the same dislocation-mediated mechanism as in the Au nanowires ( Supplementary Fig. S11 ). This result indicates that the dislocation-originated formation of SFT is a general deformation mechanism applicable to a broad class of FCC metals and alloys with medium to low stacking fault energies under mechanical loading. On the basis of the above discussions, it can be concluded that SFT formation is a general plastic deformation mechanism in metallic nanocrystals and has important consequences with respect to plastic deformation at small length scales. The deformation-induced formation of 3D defects has never been reported for nanocrystals. In the conventional bulk samples, SFT form mostly because of irradiation or quenching alone [3] , [4] , whereas in the nanocrystals, SFT can form directly from dislocation interactions. Moreover, the dislocation–SFT interaction is known to cause the SFT to be sheared into two defects, converted to other types of defects or structurally destroyed [13] , [18] , [19] , [20] , [21] . However, our work also reveals that the SFT can interact with a group of dislocations nucleated from the surface, resulting in the migration of SFT in a small and confined volume without any change in its shape and size. Such migration (that is, displacive movement) of SFT can be attributed to the active operation of surface dislocation sources that is promoted by the high stress, large image force and abundant surface nucleation sites associated with the small crystal size, while it would be rare to achieve these conditions necessary for the SFT migration in the bulk. These unusual phenomena represent the novel deformation mechanisms at the nanoscale level, and their potential effects on the strength, hardening and fracture warrant further study in the future. In summary, in situ HRTEM experiments are conducted to directly visualize the atomic-scale, dynamic evolution of a novel defect structure—dislocation-originated SFT—in Au nanocrystals. Our work for the first time discovers the formation and the dynamics of a 3D crystalline defect in small-volume nanocrystals, which has an important role in the plasticity at small length scales. These results reveal a novel deformation mechanism of dislocation interaction inside the confined volume of nanocrystals. Our work has significant implications on understanding the deformation behaviours of nanocrystals, including plastic yielding, strain hardening, ductility, size effects, and so on, which will motivate further experimental and modelling investigations of dislocation interactions and the formation of higher-order defects in small-sized materials. On the other hand, our discovery also provides an example of the deformation-induced and dislocation-originated formation mechanism of SFT in contrast to the conventional wisdom of vacancy-originated SFT, which thus expands the fundamental knowledge of 3D volume defects in small-sized, non-irradiated materials. A more detailed understanding of various factors affecting the formation of SFT warrants further study in the future. Sample Preparation and In Situ Tensile Deformation The Au nanowires were synthesized by the method reported in a recent publication [43] . The growth direction of as-synthesized Au nanowires is along the [111] direction, with few TBs parallel to the cross-section of nanowires. The tensile experiments were performed inside a FEI Tecnai F30 field emission gun TEM equipped with a Nanofactory TEM–scanning tunnelling microscope (STM) system. A charge-coupled device camera was used to record the images and videos at two frames per s. The Au nanowires were attached to an Au rod with silver paint, serving as one end of the Nanofactory TEM–STM platform. A piezo-controlled Au STM probe was used as the other end of the platform. During experiments, the Au nanowires were tilted into the [1 0] zone axis and loaded along the [111] direction. Before tensile testing, the Au probe was connected with an Au nanowire by amorphous carbon deposition at the contact area to form a strong contact. Moreover, several samples with [111] or other loading directions were made by cold welding, same as the method used in by Zheng et al . [28] . During the cold-welding process, the forward speed of the piezo-controlled Au STM probe is about 1~2 nm s −1 , whereas the linear size of the deformation-affected volume by cold welding is about 10 nm; thus the strain rate of the cold-welding process is estimated to be on the order of 0.1 s −1 . Subsequently, the tensile deformation was conducted by retracting the Au probes with the estimated strain rate of 10 −3 s −1 . The method for determining the dislocation types in HRTEM images has been discussed by Zheng et al . [28] MD simulations 3D MD simulations were carried out using LAMMPS [44] . We use the Embedded Atom Method potential developed by Grochola et al . [45] to account for the many-body interactions between Au atoms. The Au nanowires simulated are aligned along the [111] direction, along which periodic boundary condition is applied. The nanowires are geometrically cut in double conical shape of length 28.26 nm, instead of perfectly cylindrical ones; the diameters of the largest and smallest cross-sections are 6 and 4 nm, respectively. This is performed with the motivation of utilizing the stress concentration at the neck to promote sequential dislocation nucleation events instead of a large number of simultaneous nucleation events as would otherwise be observed in perfectly cylindrical single-crystal specimens. The nanowires are simulated with temperature T =1 K and loaded at a constant strain rate of 10 7 s −1 . The SFs in Figs 2 , 5d–h are visualized by colouring the atoms based on the centro-symmetry parameters, while Fig. 3 is based on the coordination numbers [46] . Figure 2e is plotted by reducing the atom sizes so as to obtain the projected images of atoms on the white background of the paper, resembling the HRTEM image. To study the size effect, MD simulations are also carried out on a larger Au nanowire with the diameters of the largest and smallest cross-sections being 10 and 6 nm, respectively. The generality of the SFT formation mechanism is verified by MD simulations of Cu nanowire. The simulation methodology and the geometry of the Cu nanowire are similar to those of Au nanowires. A recent Embedded Atom Method potential is used for Cu [47] . How to cite this article: Wang, J. W. et al . Atomic-scale dynamic process of deformation-induced stacking fault tetrahedra in gold nanocrystals. Nat. Commun. 4:2340 doi: 10.1038/ncomms3340 (2013).